DELLA-mediated gibberellin signalling regulates Nod factor signalling and rhizobial infection Legumes develop symbiotic interactions with rhizobial bacteria to form nitrogen-fixing nodules. Bacterial Nod factors (NFs) and plant regulatory pathways modulating NF signalling control rhizobial infections and nodulation efficiency. Here we show that gibberellin (GA) signalling mediated by DELLA proteins inhibits rhizobial infections and controls the NF induction of the infection marker ENOD11 in Medicago truncatula . Ectopic expression of a constitutively active DELLA protein in the epidermis is sufficient to promote ENOD11 expression in the absence of symbiotic signals. We show using heterologous systems that DELLA proteins can interact with the nodulation signalling pathway 2 (NSP2) and nuclear factor-YA1 (NF-YA1) transcription factors that are essential for the activation of NF responses. Furthermore, MtDELLA1 can bind the ERN1 (ERF required for nodulation 1) promoter and positively transactivate its expression. Overall, we propose that GA-dependent action of DELLA proteins may directly regulate the NSP1/NSP2 and NF-YA1 activation of ERN1 transcription to regulate rhizobial infections. The architecture of the root system plays a crucial role in the adaptation of plant growth to environmental settings, and is consequently a key trait to maintain crop yield in response to fluctuating extrinsic conditions. Legumes, in addition to root branching through lateral roots, can develop symbiotic interactions with soil bacteria, collectively referred to as rhizobia to form another secondary root organ, the nitrogen-fixing nodule [1] . Root nodule development is initiated by a reciprocal and specific chemical dialogue between the two symbionts. Flavonoids secreted in the rhizosphere by host legume roots induce specific rhizobia to produce signalling molecules called Nod factors (NFs) [2] , [3] . The perception of NFs in the epidermis is the first step to trigger the bacterial infection of roots, eliciting root hair deformation. Tubular cell wall ingrowths containing rhizobia, called infection threads, are then formed in curled root hairs. Simultaneously, cells in root inner layers re-enter the cell cycle, giving rise to a nodule primordium. In temperate legumes such as M. truncatula , pericycle, endodermis and inner cortical cell divisions are induced [4] . Infection threads grow across the different root outer cell layers and subsequently ramify in the cortex. Bacteria are then released into the cells of nodule primordia, which will subsequently emerge from the root [5] , [6] . In M. truncatula , a persistent meristem is established at the nodule apex, allowing an indeterminate growth. Below the nodule meristem (zone I), cells elongate and are infected by rhizobia (II), and differentiate in the central nitrogen-fixing zone (III), where bacterial and plant cells co-differentiate to fix the atmospheric nitrogen and to assimilate the ammonium produced, respectively [7] . Signalling pathways required for nitrogen-fixing symbiotic nodulation have been deciphered in the last decades [3] . Bacterial NF signals are first recognized in the root epidermis by receptor-like kinases containing LysM motives, activating a signalling cascade comprising nuclear calcium spiking. Calcium spiking is decoded by a calcium/calmodulin-dependent kinase named DMI3 (does not make infection 3) in M. truncatula , leading to the induction of nuclear transcriptional regulators essential to coordinate the expression of genes associated to rhizobial infection. Among these transcription factors, nodulation signalling pathway 1 (NSP1) and 2 (NSP2), nuclear factor-YA1 (NF-YA1), ethylene response factor required for nodulation 1 (ERN1) and nodule inception proteins are involved in the transcriptional activation of the infection marker ENOD11 in the epidermis [8] , [9] , [10] , [11] , [12] , [13] , [14] , [15] , [16] . A recent model proposes that NF-YA1 expression is NF-induced depending on DMI3 and nodule inception, and can activate ENOD11 expression in response to NFs through the regulation of ERN1 expression [15] , possibly within the same transcriptional complex as NSP1 and NSP2. This suggests that NSP1/NSP2 and NF-YA1 act synergistically to activate ERN1 expression. In addition, NSP1 binds directly to the ENOD11 promoter and this association requires NSP2 (ref. 16 ). Overall, this suggests that NSP1/NSP2, NF-YA and ERN1 act in combination to regulate the expression of early infection markers, such as ENOD11 with the appropriate spatial and temporal patterns. Beside bacterial NFs, several plant cues control nodulation progression, including phytohormones [17] . Studies based either on gain-of-function or loss-of-function mutations in a cytokinin receptor, highlight the essential role of this phytohormone in nodulation [18] , [19] , [20] , [21] . Mutations in the CRE1 (cytokinin response 1) cytokinin receptor, notably abolish the ability of rhizobia to regulate polar auxin transport locally in roots, which is correlated to the induction of nodule organogenesis [21] , [22] . In addition, this pathway directly regulates the expression of early nodulation genes such as NSP2 that is critical for bacterial NF signalling and symbiotic nodule formation [10] , [23] . Other hormones, such as ethylene and abscisic acid negatively regulate NF signalling and nodule formation [24] , [25] , [26] . In M. truncatula , the ethylene-insensitive sickle/ein2 (ethylene-insensitive 2) mutant exhibits an exaggerated number of rhizobial infection events (IEs) and a dominant-negative ABA-insensitive abi1 (abscisic acid insensitive 1) mutant is hyperinfected, as well as hypernodulating. Gibberellins (GAs) also regulate symbiotic nodulation, even though depending on plant species, positive or negative roles were reported. Indeed, the pea GA-deficient na mutant showed a decreased nodulation that was restored by an exogenous GA application, suggesting a requirement of GA in nodule initiation [27] , [28] , [29] . However, in contrast to low GA concentrations (0.001 and 1 μM), exogenous treatments with a higher GA concentration (1 mM) suppressed nodulation, indicating that a positive or a negative role of GA may exist and that a tight control of GA concentration is required [29] . In addition, the la cry constitutively active GA signalling mutant forms fewer nodules than wild-type pea plants [28] . In Lotus japonicus , exogenous GA applications (1 or 0.1 μM) or overexpression of a gain-of-function SLEEPY1 , a GA- signalling gene, resulted in an inhibition of nodulation, suppressing both epidermal infections and nodule organogenesis in the cortex [30] . Finally, in the M. truncatula model, no comprehensive data are available to explain GA functions in nodulation. Interestingly, a negative role of GA has recently been reported in rhizobial and arbuscular mycorrhizal symbioses, which are evolutionary related [31] , using a GA signalling loss-of-function della1 della2 double mutant [32] . The current model for GA signalling is that bioactive GAs are perceived by a soluble GID1 (gibberellin-insensitive dwarf-1) receptor that can interact with DELLA proteins [33] . Upon GA binding, DELLA proteins will be degraded by the proteasome through the SCF (SLY/GID2) E3 ubiquitin ligase complex. The N-terminal region of DELLA proteins contains two conserved amino-acid motives, DELLA and TVHYNP, which are essential for their interaction with the GA–GID1 complex and subsequent degradation by the proteasome pathway. The C-terminal region of DELLA proteins contains a GRAS domain (named after the founding members gibberellic-acid insensitive (GAI)/repressor of GAI (RGA)/scarecrow (SCR)) that has a putative transcriptional regulatory function [33] , [34] , [35] , [36] . Depending on their ability to interact physically with different transcription factors, DELLA proteins were initially described as repressors of GA responses even though a function of the DELLA as transactivation factors was more recently proposed [33] , [37] , [38] . In this study, we show that GAs negatively regulate M. truncatula nodulation and rhizobial infections depending on DELLA proteins. Indeed, the MtDELLA1 protein that is sufficient to promote ENOD11 expression in the epidermis can interact with the critical NF signalling factors NSP2 and NF-YA1 in heterologous systems, and activate the expression of ERN1 . This suggests a model where GA can directly regulate the NF induction of ENOD11 expression and rhizobial infections, depending on DELLA-transcriptional complexes. GAs negatively regulate nodulation in M. truncatula To investigate the role of GA during symbiotic nodulation in M. truncatula , we first assessed the effect of exogenous applications of GA 3 (from 0.001 to 1 μM) or of the GA biosynthesis inhibitor paclobutrazol (PAC; from 0.01 to 1 μM) on nodule formation ( Supplementary Fig. 1a,b ). Nodule number was decreased in the presence of exogenous GA 3 compared with the untreated condition, as a trend for lower GA concentrations (0.001 and 0.01 μM) and significantly for higher concentrations (0.1 and 1 μM; Supplementary Fig. 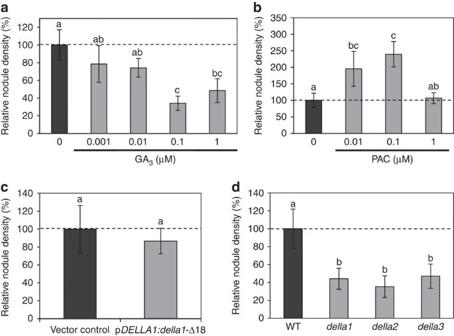Figure 1: Gibberellins regulateM. truncatulanodulation depending on DELLA proteins. (a,b) Relative nodule density (nodule number per mg of root dry weight) ofM. truncatulaplants treated with GA3(a) or PAC (b) at different concentrations. (c) Relative nodule density inM. truncatularoots expressing a dominant-active DELLA protein (pMtDELLA1:della1-Δ18) or the empty vector control. (d) Relative nodule density (nodule number per mg of root dry weight) of the threedellamutants. Results are shown as percentages relatively to the untreated control (a,b,d) or to the empty vector control (c). Quantifications were performed 21 days post inoculation withS. meliloti(strain 1021). Dotted lines indicate a ratio of 100%. Error bars represent confidence intervals (α=0.05,n>15 plants per condition), and letters indicate significant differences based on a Kruskal and Wallis test (α<0.05) for (a,b,d), and a Mann–Whitney test (α<0.05) forc. One representative example out of three biological replicates is shown. 1a ; Supplementary Table 1 ). Conversely, GA-inhibitory PAC treatments led to a significant increase in nodule number at 0.01 and 0.1 μM concentrations, but not at 1 μM ( Supplementary Fig. 1b ; Supplementary Table 1 ). These results therefore point towards a negative role of GA in nodulation, even though the absence of effect of the highest PAC concentration tested suggests that a fine control of GA levels is required to allow an efficient nodulation. As GAs are known to regulate the plant growth [33] , we characterized root and shoot phenotypes of plants treated with the different GA 3 or PAC concentrations described above, to exclude that the nodulation phenotypes previously observed were an indirect effect of the altered shoot and root development ( Supplementary Fig. 2a–c ; Supplementary Table 1 ). As expected, the shoots of GA-treated plants displayed increased internode lengths ( Supplementary Fig. 2a ). Primary root length and root dry weight of plants treated with GA 3 concentrations ranging from 0.01 to 1 μM were slightly but significantly reduced compared with untreated plants ( Supplementary Fig. 2a,b ; Supplementary Table 1 ). Conversely, PAC treatments led to a significant increase in root length and root dry weight at 0.01 and 0.1 μM, whereas no significant change was detected at 1 μM ( Supplementary Fig. 2c ; Supplementary Table 1 ). These data suggest that GAs negatively regulate M. truncatula root growth and again suggest that a fine control of GA levels is required for this regulation. Similarly, shoot phenotypes were analysed and revealed that applications of GA 3 significantly decrease shoot dry weight at high GA 3 concentrations (0.01–1 μM) ( Supplementary Table 1 ). In contrast, PAC treatments did not induce any significant effect on shoot dry weight ( Supplementary Table 1 ). To evaluate the contribution of these GA-induced developmental phenotypes on the nodulation phenotype, we then determined nodule densities, corresponding to the number of nodule either per mg of root dry weight or of shoot dry weight ( Fig. 1a,b ; Supplementary Table 1 ). Both nodule densities were decreased in the presence of exogenous GA 3 compared with the untreated condition, as a trend for lower GA concentrations (0.001 and 0.01 μM) and significantly for higher concentrations (0.1 and 1 μM; Fig. 1a ; Supplementary Table 1 ). PAC treatments led to a significant increase in nodule densities at 0.01 and 0.1 μM ( Fig. 1b ; Supplementary Table 1 ). Altogether, these results indicate that the observed negative role of GAs in nodulation can be identified independently of shoot and root growth phenotypes. Figure 1: Gibberellins regulate M. truncatula nodulation depending on DELLA proteins. ( a , b ) Relative nodule density (nodule number per mg of root dry weight) of M. truncatula plants treated with GA 3 ( a ) or PAC ( b ) at different concentrations. ( c ) Relative nodule density in M. truncatula roots expressing a dominant-active DELLA protein (p MtDELLA1 : della1- Δ18) or the empty vector control. ( d ) Relative nodule density (nodule number per mg of root dry weight) of the three della mutants. Results are shown as percentages relatively to the untreated control ( a , b , d ) or to the empty vector control ( c ). Quantifications were performed 21 days post inoculation with S. meliloti (strain 1021). Dotted lines indicate a ratio of 100%. Error bars represent confidence intervals ( α =0.05, n >15 plants per condition), and letters indicate significant differences based on a Kruskal and Wallis test (α<0.05) for ( a , b , d ), and a Mann–Whitney test ( α <0.05) for c . One representative example out of three biological replicates is shown. Full size image GA regulation of nodulation depends on DELLA proteins As DELLA proteins are central repressors of GA-dependent responses [33] , [34] , [35] , [36] , we hypothesized that GAs could control the nodule formation depending on DELLAs as suggested by Floss et al . [32] Three DELLA genes are present in the M. truncatula genome: MtDELLA1 (Medtr3g065980, M. truncatula genome v4.0 database; http://jcvi.org/medicago/ ), MtDELLA2 (contig_52215, NCBI database; http://www.ncbi.nlm.nih.gov ) and MtDELLA3 (contig_55897, NCBI database; http://www.ncbi.nlm.nih.gov ). The encoded proteins MtDELLA1 and MtDELLA2 are, respectively, most closely related to the Arabidopsis DELLA proteins AtRGL1–3 and AtRGA/AtGAI, and are the closest relatives of the pea DELLA proteins PsLA and PsCRY [32] . The M. truncatula MtDELLA3 protein is more divergent compared with Arabidopsis and pea DELLAs, containing a non-canonical DGLLA domain [32] . The expression patterns of the three MtDELLA genes, based on the M. truncatula Gene Expression Atlas (MtGEA database, http://mtgea.noble.org/v3/ ; ref. 39 ), revealed that MtDELLA1 and MtDELLA2 have similar transcript levels in roots and nodules, and that MtDELLA3 has an overall weaker expression level. In addition, the three MtDELLA genes do not show any strong transcriptional regulation in response to bacterial NFs [32] ( Supplementary Fig. 3a,b ; ref. 40 ). Laser dissection of different nodule zones associated with RNAseq revealed a preferential expression of the three DELLA genes in the meristematic zone (I), and a lower expression of MtDELLA1 and MtDELLA2 in the differentiation/infection zone (II; SYMBIMICS database, https://iant.toulouse.inra.fr/symbimics/ ; ref. 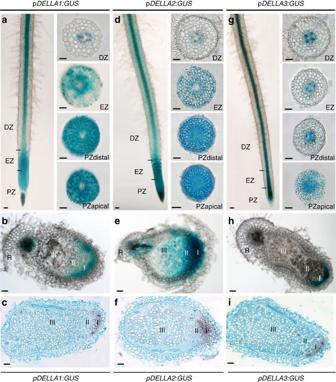Figure 2:DELLAexpression patterns inM. truncatularoots inoculated with rhizobium and symbiotic nodules. Histochemical analysis of GUS activity ofMtDELLAtranscriptional fusions in roots (1 day post inoculation (dpi) withS. meliloti) and nodules (21 dpi). Whole roots or 40 μm thick transversal root and nodule sagittal sections ofMtDELLA1:GUS(a,b),MtDELLA2:GUS(d,e) andMtDELLA3:GUS(g,h) are shown. (c,f,i) arein situhybridizations ofMtDELLA1(c),MtDELLA2(f) andMtDELLA3(i) transcripts in 40 μm thick nodule longitudinal sections. Root zones are described as follows: DZ, differentiation zone; EZ, elongation zone; PZ, proliferation zone. Nodule zones are described as follows: I, meristem; II, infection/differentiation zone; III, nitrogen-fixation zone (according to Vasseet al.7); R, root. Scale bars, 100 μm. One representative example out ofn=20 independent roots for histochemical analysis of GUS activity andn=5 nodules forin situhybridization is shown. 41 ; Supplementary Table 2 ). The spatial expression pattern of the three MtDELLA genes was investigated using MtDELLA promoter:GUS (β- glucuronidase) transcriptional fusions. Under non-symbiotic and symbiotic conditions (1 day after inoculation with Sinorhizobium meliloti ), the expression of the three MtDELLA genes was detected in the rhizobial infection zone (located above the root apical meristem, in the region where root hairs differentiate), in the root stele and cortex, and additionally in the epidermis for MtDELLA1 and MtDELLA2 ( Fig. 2a,d,g ; Supplementary Fig. 3c–e ). The epidermal expression of MtDELLA1 and MtDELLA2 is consistent with transcriptomic results recently obtained by Breakspear et al . [40] ( Supplementary Fig. 3b ). In differentiated nitrogen-fixing nodules, the DELLA genes were mainly expressed in the meristematic zone I ( Fig. 2b,e,h ), in accordance with laser dissection transcriptomic data ( Supplementary Table 2 ). This spatial expression pattern was independently validated using in situ hybridization ( Fig. 2c,f,i ). Figure 2: DELLA expression patterns in M. truncatula roots inoculated with rhizobium and symbiotic nodules. Histochemical analysis of GUS activity of MtDELLA transcriptional fusions in roots (1 day post inoculation (dpi) with S. meliloti ) and nodules (21 dpi). Whole roots or 40 μm thick transversal root and nodule sagittal sections of MtDELLA1:GUS ( a , b ), MtDELLA2:GUS ( d , e ) and MtDELLA3:GUS ( g , h ) are shown. ( c , f , i ) are in situ hybridizations of MtDELLA1 ( c ), MtDELLA2 ( f ) and MtDELLA3 ( i ) transcripts in 40 μm thick nodule longitudinal sections. Root zones are described as follows: DZ, differentiation zone; EZ, elongation zone; PZ, proliferation zone. Nodule zones are described as follows: I, meristem; II, infection/differentiation zone; III, nitrogen-fixation zone (according to Vasse et al . [7] ); R, root. Scale bars, 100 μm. One representative example out of n =20 independent roots for histochemical analysis of GUS activity and n =5 nodules for in situ hybridization is shown. Full size image To determine the involvement of DELLA proteins in symbiotic nodulation, we first expressed from the MtDELLA1 endogenous promoter a dominant version of the MtDELLA1 protein deleted of its DELLA domain ( della1 -Δ18; ref. 32 ), which is therefore insensitive to GA-dependent degradation. The expression of the della1 -Δ18 gene did not reveal any significant nodulation phenotype ( Fig. 1c ; Supplementary Fig. 1c ), even though the expression of the transgene was clearly detected ( Supplementary Fig. 1f ). Second, as the three DELLA genes are expressed in similar regions in roots and/or nodules, suggesting a potential functional redundancy ( Fig. 2 ), we identified Tnt1 insertional mutants affecting these three genes. della1, della2 and della3 mutants displayed shoot phenotypes typical of mutants having constitutively active GA responses, namely a longer stem and an early flowering phenotype [32] , [33] ( Supplementary Fig. 4 ). Primary root length, and root and shoot dry weights of the three della mutants, however, did not significantly differ from wild-type plants ( Supplementary Fig. 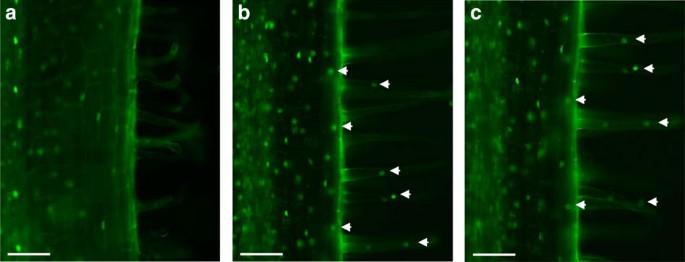Figure 3: Nuclear localization of the MtDELLA1 protein under non-symbiotic and symbiotic conditions. Rhizobium infection zones ofM. truncatularoots expressing the pMtDELLA1:GFP-della1-Δ18 construct are shown under control conditions (untreated,a), after a 6 h 10−9M Nod factors (NF) treatment (b) or 1 day after inoculation withS. meliloti(strain 1021) (c). White arrowheads indicate GFP signals in the nuclei of epidermal cells, including in root hairs. Scale bars, 100 μm. 2d ; Supplementary Table 3 ). After S. meliloti inoculation, the three della mutants showed significantly reduced nodule numbers and densities ( Fig. 1d ; Supplementary Fig. 1d,e ; Supplementary Table 3 ). Complementation assays of the three della mutants were performed using the respective pMtDELLAx:DELLAx-HA translational fusions, and both nodule number and density were restored ( Supplementary Fig. 5 ). The identified nodulation phenotypes of single della mutant are therefore consistent with those obtained by Floss et al . [32] , with a della1 della2 double mutant. Taken together, these results suggest that in M. truncatula , GAs play a negative role in nodule formation depending on a DELLA signalling pathway. MtDELLA1 symbiotic nuclear localization in the root epidermis To determine the subcellular localization of the three MtDELLA proteins, a transient expression assay in Nicotiana benthamiana was first used to ectopically express MtDELLA-GFP (green fluorescent protein) translational fusions from the 35S-CaMV promoter. The three MtDELLA-GFP fusions were detected in the nucleus, as expected from data gained in Arabidopsis ( Supplementary Fig. 3f ; ref. 42 ). To monitor DELLA subcellular localization in M. truncatula roots, we used the same translational fusions, but no GFP signal could be detected, either using the strong constitutive 35S-CaMV promoter or the endogenous MtDELLA1 promoter, in agreement with data obtained by Floss et al . [32] To overcome the fast DELLA protein turn over due to their continuous degradation by the proteasome pathway [43] , we used an N-terminal GFP translational fusion with the GA-insensitive della1 -Δ18 variant expressed from the MtDELLA1 promoter, previously used and functionally validated in M. truncatula roots [32] . This stabilized GFP- della1 -Δ18 fusion was detected in the nuclei of cortical and stele cells ( Fig. 3a ). Interestingly, in response to NFs ( Fig. 3b ) or S. meliloti inoculation ( Fig. 3c ), the GFP- della1 -Δ18 fusion was additionally detected in the nuclei of epidermal cells, notably in the rhizobial susceptible zone. These results indicate that at least the MtDELLA1 GA signalling factor is present in the epidermis under symbiotic conditions. Figure 3: Nuclear localization of the MtDELLA1 protein under non-symbiotic and symbiotic conditions. Rhizobium infection zones of M. truncatula roots expressing the p MtDELLA1 :GFP- della1- Δ18 construct are shown under control conditions (untreated, a ), after a 6 h 10 −9 M Nod factors (NF) treatment ( b ) or 1 day after inoculation with S. meliloti (strain 1021) ( c ). White arrowheads indicate GFP signals in the nuclei of epidermal cells, including in root hairs. Scale bars, 100 μm. Full size image GA and DELLAs regulate rhizobial infections in the epidermis To determine if bacterial infection in the epidermis is affected by the GA signalling pathway, we used a LacZ -expressing S. meliloti strain that allows visualization and quantification of IEs ( Fig. 4 ). Exogenous GA 3 application drastically reduced IE density and accordingly, in the three della mutants, IE density was also strongly decreased ( Fig. 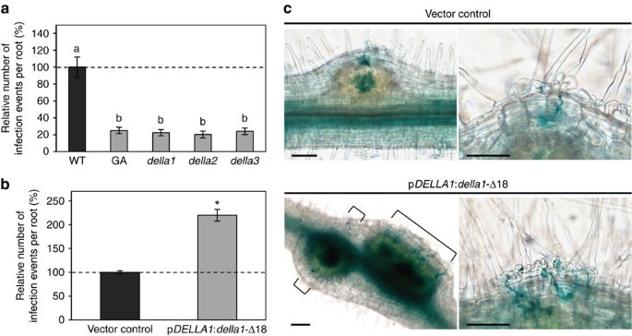Figure 4: Gibberellins regulateM. truncatulainfection depending on DELLA proteins. (a) Quantification of infection events per root in wild type (WT), with or without GA3(1 μM) or indellamutants. Results are shown as percentages relatively to the WT untreated control. (b) Relative number of infection events in roots expressing the pMtDELLA1:della1-Δ18 construct. Results are shown as percentages relatively to the empty vector used as control. (c) Representative images of nodule primordia (left panels) in roots expressing the empty vector (top) or in roots expressing the pMtDELLA1:della1-Δ18 construct (bottom). Details of infected root hairs are shown in right panels. Square brackets indicate infection threads. Scale bars, 100 μm. In (a,b), dotted lines indicate a ratio of 100%. In all cases, quantifications were performed 7 days post inoculation with aS. melilotiexpressing aLACZreporter. Error bars represent confidence intervals (α=0.05,n>10 plants), and letters and star indicate significant differences based on a Kruskal and Wallis test (α<0.05) foraand a Mann–Whitney test (α<0.05) forb. One representative example out of two biological replicates is shown. 4a ; Supplementary Table 4 ). In addition, transgenic roots expressing the della1- Δ18 variant showed an increased IE density, even though no nodulation phenotype was previously observed ( Fig. 1c ; Fig. 4b,c ). This result again suggests that a fine regulation of GA levels is needed to allow an efficient nodulation. Overall, these results indicate that GAs negatively regulate IEs by suppressing DELLA activity. Figure 4: Gibberellins regulate M. truncatula infection depending on DELLA proteins. ( a ) Quantification of infection events per root in wild type (WT), with or without GA 3 (1 μM) or in della mutants. Results are shown as percentages relatively to the WT untreated control. ( b ) Relative number of infection events in roots expressing the p MtDELLA1 : della1- Δ18 construct. Results are shown as percentages relatively to the empty vector used as control. ( c ) Representative images of nodule primordia (left panels) in roots expressing the empty vector (top) or in roots expressing the p MtDELLA1:della1 -Δ18 construct (bottom). Details of infected root hairs are shown in right panels. Square brackets indicate infection threads. Scale bars, 100 μm. In ( a , b ), dotted lines indicate a ratio of 100%. In all cases, quantifications were performed 7 days post inoculation with a S. meliloti expressing a LACZ reporter. Error bars represent confidence intervals ( α =0.05, n >10 plants), and letters and star indicate significant differences based on a Kruskal and Wallis test ( α <0.05) for a and a Mann–Whitney test ( α <0.05) for b . One representative example out of two biological replicates is shown. Full size image To pinpoint molecular mechanisms that could explain this phenotype, we analysed the effect of GAs on the expression of one of the earliest NF-induced infection marker: ENOD11 (ref. 8 ). Transgenic plants expressing a p ENOD11:GUS transcriptional fusion were treated with NF for 3 h, with or without a 3 h GA 3 pre-treatment. As previously described [8] , the NF-induced ENOD11 expression was detected in epidermal cells of the rhizobial infection zone ( Fig. 5a ). Interestingly, a pre-treatment with GA 3 inhibited the NF induction of ENOD11 ( Fig. 5a ). To independently and quantitatively confirm this result, the expression of ENOD11 was determined by real-time PCR with reverse transcription (RT–PCR) in roots challenged with the same treatments. The efficiency of the GA 3 treatment was determined by monitoring the expression of a GA catabolic ( GA2ox ) and of a GA biosynthetic ( GA20ox ) gene, which are, respectively, up- and downregulated by the exogenous GA 3 treatment, as a result of a negative feedback (ref. 44 ; Fig. 5b ). As previously observed, the NF-induced expression of ENOD11 was drastically reduced in GA 3 pre-treated roots ( Fig. 5b ). Because MtDELLA1 was detected in the nuclei of epidermal cells in the rhizobial susceptible zone under symbiotic conditions ( Fig. 3b,c ), and because the expression of the della1- Δ18 variant increased IE density ( Fig. 4b ), we tested if the NF induction of ENOD11 depended on MtDELLA1. The NF regulation of ENOD11 was strongly reduced in the della1 mutant ( Fig. 5c ). Together, these results indicate that in agreement with the previously observed infection and nodulation phenotypes, the early NF-dependent ENOD11 expression is rapidly regulated by GAs depending at least on MtDELLA1. 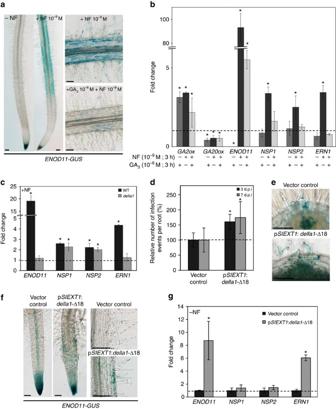Figure 5: Gibberellins regulate rhizobial infection andENOD11expression depending on MtDELLA1 activity in the epidermis. (a) Histochemical localization of GUS activity in 7-day- old transgenic seedlings expressing the rhizobial infection markerpENOD11:GUSafter a NF (10−9M) treatment and with or without a GA3(1 μM) pre-treatment. (b) Expression ofGA2ox, GA20ox, NSP1, NSP2,ERN1andENOD11in WT roots after a NF (10−9M) treatment, and with or without a GA3(1 μM) pre-treatment. (c) Expression of theENOD11infection marker and ofNSP1, NSP2andERN1after a NF (10−8M) treatment in the WT and indella1mutant roots. (d) Relative number of infection events in pSlEXT1:della1-Δ18 roots, at 3 and 7 days post inoculation withS. meliloti(strain 2011) expressing theLACZreporter. Results are shown as percentages relatively to the empty vector control. (e) Representative images of infection threads visualized by staining ofS. meliloti(strain 2011) expressing theLACZreporter in roots transformed with the vector control (top) or the pSlEXT1:della1-Δ18 (bottom) construct. (f) Histochemical localization of GUS activity in transgenic roots expressing pENOD11:GUS, transformed with the empty vector control or the pSlEXT1:della1-Δ18 construct. Details of root hairs are shown in right panels. (g) Expression ofENOD11, NSP1, NSP2andERN1in non-inoculated roots expressing pSlEXT1:della1-Δ18 or the vector control. Inb,candg, transcript levels are normalized relatively to untreated control roots to show fold changes and the dotted line indicates a ratio of 1. Ind, results are shown as percentages relatively to the empty vector control and dotted line indicates a ratio of 100%. Error bars represent s.d. inb,candg, and confidence intervals (α=0.05,n>15 plants per condition) ford. In all cases, the asterisks indicate significant difference compared with the control based on a Mann–Whitney test (α<0.05). One representative example out of two biological replicates is shown. Scale bars, 100 μm (a,e). Figure 5: Gibberellins regulate rhizobial infection and ENOD11 expression depending on MtDELLA1 activity in the epidermis. ( a ) Histochemical localization of GUS activity in 7-day- old transgenic seedlings expressing the rhizobial infection marker pENOD11 : GUS after a NF (10 −9 M) treatment and with or without a GA 3 (1 μM) pre-treatment. ( b ) Expression of GA2ox, GA20ox, NSP1, NSP2 , ERN1 and ENOD11 in WT roots after a NF (10 −9 M) treatment, and with or without a GA 3 (1 μM) pre-treatment. ( c ) Expression of the ENOD11 infection marker and of NSP1, NSP2 and ERN1 after a NF (10 −8 M) treatment in the WT and in della1 mutant roots. ( d ) Relative number of infection events in p SlEXT1 : della1- Δ18 roots, at 3 and 7 days post inoculation with S. meliloti (strain 2011) expressing the LACZ reporter. Results are shown as percentages relatively to the empty vector control. ( e ) Representative images of infection threads visualized by staining of S. meliloti (strain 2011) expressing the LACZ reporter in roots transformed with the vector control (top) or the p SlEXT1 : della1- Δ18 (bottom) construct. ( f ) Histochemical localization of GUS activity in transgenic roots expressing p ENOD11 : GUS , transformed with the empty vector control or the p SlEXT1 : della1 -Δ18 construct. Details of root hairs are shown in right panels. ( g ) Expression of ENOD11, NSP1, NSP2 and ERN1 in non-inoculated roots expressing p SlEXT1 : della1 -Δ18 or the vector control. In b , c and g , transcript levels are normalized relatively to untreated control roots to show fold changes and the dotted line indicates a ratio of 1. In d , results are shown as percentages relatively to the empty vector control and dotted line indicates a ratio of 100%. Error bars represent s.d. in b , c and g , and confidence intervals ( α =0.05, n >15 plants per condition) for d . In all cases, the asterisks indicate significant difference compared with the control based on a Mann–Whitney test ( α <0.05). One representative example out of two biological replicates is shown. Scale bars, 100 μm ( a , e ). Full size image To further test whether MtDELLA1 has a role in symbiosis in the epidermis, the della1 -Δ18 dominant-active protein was expressed from a p SlEXT1 promoter ( Solanum lycopersicum extensin1), previously demonstrated to be specifically active in the epidermis of M. truncatula roots [45] . Either 3 or 7 days after inoculation with S. meliloti , IE density was significantly increased in these roots ( Fig. 5d,e ; Supplementary Table 4 ), indicating that the ectopic expression of a dominant version of MtDELLA1 in the epidermis is sufficient to promote rhizobial infection. Accordingly, the ectopic expression of della1 -Δ18 in the epidermis of stable transgenic plants expressing the p ENOD11:GUS transcriptional fusion revealed an activation of the ENOD11 promoter in epidermal cells of the rhizobial infection zone in the absence of rhizobia or NFs ( Fig. 5f ). This result was independently and quantitatively confirmed by real-time RT–PCR ( Fig. 5g ), indicating that the dominant active form of a DELLA protein expressed in the epidermis is sufficient to spontaneously activate a symbiotic infection pathway related to ENOD11 . This suggests that the GA regulation of symbiotic infections and NF signalling depends on the cell autonomous action in the root epidermis of at least MtDELLA1. MtDELLA1 interacts with NSP2 and NF-YA1 and activate ERN1 As GAs inhibit the NF induction of the ENOD11 symbiotic infection marker, the expression of which directly depends on the previously identified NF signalling genes NSP1 , NSP2 and ERN1 (refs 10 , 11 , 12 , 13 , 14 ), we then investigated if GAs could affect their expression. The NF induction of NSP1, NSP2 and ERN1 was inhibited by a GA 3 pre-treatment ( Fig. 5b ), suggesting that GAs negatively regulate nodulation potentially by repressing these key NF signalling genes. We therefore tested if MtDELLA1 was involved in this regulation. The NF induction of NSP1 and NSP2 expression was maintained in the della1 mutant, whereas the NF induction of ERN1 and ENOD11 was strongly reduced ( Fig. 5c ). This suggests that the MtDELLA1-dependent induction of ENOD11 expression by NFs may require activation of ERN1. Interestingly, in the absence of rhizobia or NFs, the ectopic expression of della1 -Δ18 in the epidermis previously shown to induce ENOD11 expression, was sufficient to activate ERN1 as well, but not NSP1 and NSP2 ( Fig. 5g ). These results indicate that at least MtDELLA1 is required in the epidermis to activate both ERN1 and ENOD11 expression. Accordingly, a chromatin immunoprecipitation (ChIP) experiment performed in M. truncatula roots 1 day post inoculation with rhizobium indicated that pMtDELLA1:MtDELLA1 can associate with the ERN1 promoter ( Supplementary Fig. 6 ). The NSP1/NSP2 GRAS and the NF-YA1 transcription factors have been previously shown to directly bind the ERN1 promoter to positively regulate its expression [13] , [14] , [15] , [16] . As we now demonstrated that at least MtDELLA1 is required to induce ERN1 and ENOD11 expression in response to NFs ( Fig. 5c ), and as DELLA proteins have been previously shown to interact with transcription factors [33] , we then tested if DELLA proteins were able to interact with the NSP1, NSP2 or NF-YA1 transcription factors ( Fig. 6 ). Using bimolecular fluorescence complementation (BiFC), interactions in the nuclei could be detected between the three DELLA proteins and NSP2 ( Fig. 6b ), but not NSP1 ( Fig. 6a ). As previously described [16] , the NSP1 BiFC construct revealed an interaction with NSP2 ( Fig. 6d ), indicating its functionality and thus revealing specificities among GRAS protein interactions. In addition, a nuclear interaction between the three DELLA proteins and the NF-YA1 transcription factor was detected ( Fig. 6c ). Interactions between the three DELLA proteins, and the transcription factors NSP2 and NF-YA1 were further independently confirmed by co-immunoprecipitation (Co-IP) assays in N. benthamiana leaves ( Fig. 6e,f ). As NF-YA1 and NSP2 proteins may be recovered simultaneously in a MtDELLA IP, this suggests that these protein interactions might not be exclusive ( Supplementary Fig. 7 ). Overall, these results indicate that M. truncatula DELLA proteins can interact, at least in heterologous systems, with two critical NF signalling transcription factors, NF-YA1 and NSP2, known to positively regulate the ERN1 symbiotic expression. 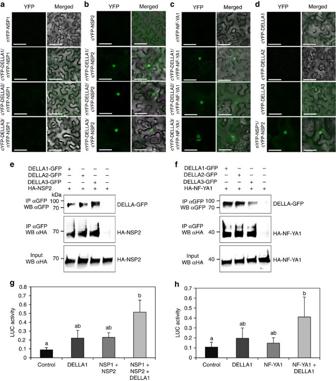Figure 6: DELLAs can interact with the NF signalling transcription factors NSP2 and NF-YA1, and MtDELLA1 can enhanceERN1transcriptional activation. (a–d). Bimolecular fluorescence complementation analysis of the interaction between nYFP-NSP1 and cYFP-MtDELLA1 to 3 (a), cYFP-NSP2 and nYFP-MtDELLA1 to 3 (b), and nYFP-NF-YA1 and cYFP-MtDELLA1 to 3 (c) inN. benthamianaleaves. The negative controls (each construct alone) are shown in the different panels, as well as the nYFP-NSP1-cYFP-NSP2-positive control (d). In all panels, YFP fluorescence alone (left) and bright-field merged images (right) are shown. Scale bars, 100 μm. (e,f) Co- immunoprecipitation of MtDELLA1-GFP, MtDELLA2-GFP or MtDELLA3-GFP proteins expressed inN. benthamianaleaves with either the HA-NSP2 protein (e) or the HA-NF-YA1 protein (f). Blots were revealed with an anti-GFP (upper panel) or an anti-HA (middle and lower panels) antibody. Inputs were used as loading controls. (g,h) Transactivation assays inA. thalianaprotoplasts of thepERN1:LUCconstruct by NSP1/NSP2 (a) or NF-YA1 (b) with or without MtDELLA1. An empty vector is used as negative control. Results represent the means of two biological replicates, error bars represent the s.e., and letters indicate significant differences (α<0.01) using a Kruskal and Wallis test. Figure 6: DELLAs can interact with the NF signalling transcription factors NSP2 and NF-YA1, and MtDELLA1 can enhance ERN1 transcriptional activation. ( a – d ). Bimolecular fluorescence complementation analysis of the interaction between nYFP-NSP1 and cYFP-MtDELLA1 to 3 ( a ), cYFP-NSP2 and nYFP-MtDELLA1 to 3 ( b ), and nYFP-NF-YA1 and cYFP-MtDELLA1 to 3 ( c ) in N. benthamiana leaves. The negative controls (each construct alone) are shown in the different panels, as well as the nYFP-NSP1-cYFP-NSP2-positive control ( d ). In all panels, YFP fluorescence alone (left) and bright-field merged images (right) are shown. Scale bars, 100 μm. ( e , f ) Co- immunoprecipitation of MtDELLA1-GFP, MtDELLA2-GFP or MtDELLA3-GFP proteins expressed in N. benthamiana leaves with either the HA-NSP2 protein ( e ) or the HA-NF-YA1 protein ( f ). Blots were revealed with an anti-GFP (upper panel) or an anti-HA (middle and lower panels) antibody. Inputs were used as loading controls. ( g , h ) Transactivation assays in A. thaliana protoplasts of the pERN1:LUC construct by NSP1/NSP2 ( a ) or NF-YA1 ( b ) with or without MtDELLA1. An empty vector is used as negative control. Results represent the means of two biological replicates, error bars represent the s.e., and letters indicate significant differences ( α <0.01) using a Kruskal and Wallis test. Full size image We then finally investigated whether MtDELLA proteins could influence the transcriptional activation of ERN1 mediated by the NSP1/NSP2 or NF-YA1 transcription factors ( Fig. 6g,h ). Interestingly, transient activation assays in Arabidopsis protoplasts revealed that the expression of a p ERN1:LUC reporter construct is significantly increased when NSP1/NSP2 ( Fig. 6g ) or NF-YA1 ( Fig. 6h ) are co-transfected with MtDELLA1 . These results suggest that at least MtDELLA1 is able to function as a transcriptional activator of ERN1 expression in protoplasts, which can potentiate the action of the NSP1/NSP2 and NF-YA1 transcription factors. Overall, based on these results, we propose that MtDELLA1 protein positively regulates the expression of ERN1 , depending on its ability to interact with key NF signalling transcription factors binding the ERN1 promoter, to subsequently regulate the ENOD11 expression and the progression of rhizobial infections. In legumes, root symbiotic nodulation is tightly and dynamically regulated to ensure that the extent of rhizobial infections, nodule number and ultimately nitrogen-fixation activity are coordinated with the availability of other soil nitrogen sources and with the carbon provided from shoots. This control is notably exerted by several plant hormones that affect different stages of symbiotic nodulation. Most plant hormones previously reported to regulate rhizobial infection and/or NF signalling in the epidermis have been described to act at or upstream of calcium spiking. For instance, ethylene, abscisic acid and jasmonic acid inhibit the rhizobial infection by negatively regulating the multiple epidermal responses [24] , [25] , [26] . Whereas ethylene and abscisic acid act in parallel pathways to regulate early infection stages, jasmonic acid and ethylene act synergistically to inhibit the nodulation, but these two hormones have an antagonistic role in the regulation of the calcium spiking [24] , [25] , [26] , [46] . This indicates that complex crosstalk between several hormones control NF signalling upstream of calcium spiking, even though molecular mechanisms involved remain unknown. Consistent with the Maekawa et al . [30] study in L. japonicus , we show in this study that the GA phytohormones play a negative role in M. truncatula nodulation at an early step of the NF signal transduction pathway, downstream of calcium spiking. This regulation may involve an interaction between the GRAS transcriptional regulators DELLA, acting in GA signalling, and the NF signalling transcription factors NSP2 and NF-YA1, highlighting potential crosstalk between these two signalling pathways. Previous studies already revealed that GAs play an important role in legume nodulation, either positive or negative depending on legume species and experimental approaches used [17] . On the one hand, in Sesbania rostrata lateral root-based nodulation, a GA biosynthesis inhibitory treatment with chlormequat chloride decreased nodulation; in pea, exogenous GA 3 applications at low concentrations (0.001 and 1 μM) increased nodulation and a 1 μM GA 3 treatment was able to rescue the reduced nodulation phenotype of the dwarf GA biosynthetic na mutant [27] , [47] . In addition, GA 3 applications in L. japonicus induced the formation of pseudo-nodule structures in the absence of rhizobia [48] . These data suggest that GAs act positively in nodulation and notably in organogenesis. On the other hand, the application of exogenous GA 3 (10 μM) inhibited root hair curling nodulation in S. rostrata and infection in L. japonicus, and a high GA 3 concentration (1 mM) decreased pea nodulation [27] , [30] , [47] . In L. japonicus , exogenous GA 3 applications ranging from 0.001 to 1 μM inhibited root nodule formation and conversely, treatments with a GA biosynthesis inhibitor increased nodule number [30] . Accordingly, a gain-of-function mutation of the L. japonicus GA signalling F-box protein SLEEPY1 (SLY1) [30] and a pea DELLA loss-of-function la cry double mutant [28] show a reduced number of nodules, indicating that the DELLA-dependent GA signalling pathway positively regulates nodulation. This suggests a negative role of GAs in nodulation, notably in rhizobial infection. Accordingly in M. truncatula, exogenous applications of GA 3 (in the same concentration range as tested in L. japonicus ) and mutation in della genes decreased the number of nodules and epidermal infections [32] (and this study), whereas low PAC concentrations increased the number of nodules and the expression of the della1 -Δ18 variant from the MtDELLA1 promoter increased the number of infections. This therefore reveals a negative role of GA and a positive role of DELLA proteins in M. truncatula nodulation and rhizobial infection. Higher PAC concentrations (1 μM) or della1 -Δ18 roots however did not lead to the formation of an increased number of nodules in M. truncatula , as it would be expected. Altogether, these data suggest that a fine-tuned GA ‘window’ is required for an efficient nodulation, which may depend on species and approaches used [17] , [27] , [28] , [29] . Several transcriptomic analyses revealed that the expression of GA metabolic genes, such as GA2ox catabolic and GA20ox biosynthetic genes, are regulated during early nodulation a few hours after rhizobium or NF application [40] , [47] , [49] , [50] (and this study), as well as in the evolutionary-related mycorrhizal endosymbiosis [51] , [52] , [53] , where a significant increase of endogenous GA levels is observed during colonization [54] . In L. japonicus , depending on GA concentrations, positive or negative effects on the expression of mycorrhizal infection genes have been observed [55] , [56] , and in pea, a GA 3 treatment decreased hyphal colonization and arbuscule formation, but increased hyphal branching in cortical cell layers [52] , [53] . These results indicate a dual function of GA in the regulation of endomycorrhiza symbioses, which is reminiscent of results obtained in symbiotic nodulation. Several recent studies also highlighted that a shared GA/DELLA regulation may exist between NF and Myc factor signalling pathways. Indeed, pea la cry and M. truncatula della1 della2 double mutants have both a drastic decrease in arbuscule formation, associated to a reduction of hyphal growth in pea, but not in M. truncatula [32] , [57] . Similarly in rice, a mutation of the OsSLR1 DELLA protein induced a severe reduction of hyphaes, arbuscules and vesicles, whereas hyphopodia formation seemed unaffected [58] . All these studies then point to a positive role of DELLA proteins in the regulation of arbuscule differentiation and/or AM colonization, as observed for nodulation and rhizobial infection. Accordingly to the transcriptomic data, in situ and GUS transcriptional fusions revealed that the three MtDELLA genes have similar expression patterns in the root rhizobial infection zone and in nodules, suggesting a potential redundancy, similarly as in Arabidopsis where the five AtDELLA proteins have partially overlapping functions [33] . Nodulation phenotypes of M. truncatula mutants affecting each of the three MtDELLA genes have a similar strength, although MtDELLA3 has a modified DELLA domain (DGLLA) and a weaker expression level than MtDELLA1 and MtDELLA2 . Noteworthy, GA-related shoot phenotypes observed in each single della mutant also have a similar strength, even though MtDELLA3 expression is weaker than MtDELLA1 and MtDELLA2 also in shoots. This may indicate that the absence of one DELLA may affect the function of the others. The nodulation phenotype of the three single della mutants reported in this study appears to be stronger than the one previously observed in a della1 della2 double mutant [32] . These discrepancies between studies may be explained by the use of different della1 mutant alleles, diverse rhizobial strains, inoculation and plant growth conditions, as well as ways to score nodulation phenotypes. Accordingly, strong GA-related shoot phenotypes observed in our study in single della mutants were not reported elsewhere [32] . Nevertheless, both studies identified a low nodulation phenotype, independently of della mutant alleles and combinations used [32] (and this study), further indicating a positive role of DELLA in M. truncatula early nodulation. Interestingly, the GFP- della1 -Δ18 translational fusion revealed a nuclear accumulation of the GFP signal in epidermal cells under symbiotic conditions, although no GFP signal was detected in the epidermis under non-symbiotic conditions. Whereas we do not exclude that a DELLA protein level below the GFP detection limit exists, an alternative interpretation would be that DELLA proteins might be recruited in the epidermis in response to rhizobium and NFs, implying that such regulation would be independent of the NSP/ERN NF signalling pathway. Strikingly, transcriptional analyses in M. truncatula also revealed that most of the NF signalling genes, such as NSP1, NSP2, ERN1 and NF-YA1 are themselves rapidly induced by NFs [10] , [12] , [13] , [14] , [15] , including in root hairs [40] . DELLAs would therefore be another example of a critical NF signalling component, which regulation depends on its own pathway, even though in the case of DELLA proteins, this regulation may involve post-transcriptional regulations. Interestingly, DELLA function in arbuscular mycorrhizal symbiosis was proposed to act non-cell autonomously from the vascular tissues and endodermis to enable arbuscule formation in a distant cortex layer, and a movement of DELLA proteins was hypothesized to explain this non-cell autonomous effect [32] . During rhizobial infection, a specific transcriptional cascade in the epidermis leads to the activation of the infection marker ENOD11 (ref. 9 ). In L. japonicus , Maekawa et al . [30] demonstrated that GAs negatively regulate the NF-induced expression of NSP1 and NSP2. Our study shows that the NF induction of the ERN1 expression, acting upstream of ENOD11 , is strongly inhibited by a GA treatment. In addition, the NF-induced ERN1 expression was lost in the della1 mutant and the ectopic expression of the stabilized dominant-active della1- Δ 18 variant in the epidermis was able, in the absence of bacterial or NF signals, to induce ERN1 expression. This indicates that the epidermal expression of MtDELLA1 under non-symbiotic conditions is sufficient to activate at the molecular level an infection-related pathway. As it was recently proposed that NSP1/NSP2 and NF-YA1 transcriptional complexes directly participate in the NF regulation of ERN1 to subsequently activate ENOD11 expression [14] , [15] , these results suggest that the induction of ERN1 expression requires MtDELLA1-dependent activation of NF-YA1 and/or NSP1/2 complexes. DELLA proteins can recruit different types of transcription factors to regulate gene expression with a high spatiotemporal specificity [33] . We show in this study that MtDELLA1, MtDELLA2 and MtDELLA3 can interact with NSP2 and NF-YA1. It should be however noted that these protein interactions were only detected in a heterologous system, and not in M. truncatula roots. We could nevertheless demonstrate in M. truncatula roots that MtDELLA1 expressed from its own promoter can bind the ERN1 promoter, and can promote its expression in an heterologous transactivation assay. Altogether, based on these results, we propose that, in addition to NSP2 and NF-YA1 transcription factors, DELLA proteins act as positive transactivation factors of ERN1 expression. Related functions were recently described in Arabidopsis and rice [33] , [37] , [38] . Indeed, while DELLA proteins were mainly considered until recently as having a repressive role, the AtRGA protein was shown to form a complex with an IDD protein (indeterminate domain) to upregulate the expression of SCL3 (scarecrow-like 3) [37] . In addition, GRAS transcription factors related to NSP2 have also recently been identified as interactors of a DELLA protein in rice [58] . As mentioned previously, GA and DELLA proteins seem to have similar functions in early rhizobial and endomycorrhizal interactions. At the molecular level, the unique rice DELLA, OsSLR1 (slender rice 1) interacts with the GRAS protein DIP1 (standing for DELLA interacting protein 1), which is positively involved in the endomycorrhiza symbiotic interaction. DIP1 interacts with another GRAS transcription factor, RAM1 (reduced arbuscular mycorrhization 1) required for the activation of the RAM2 mycorrhizal-induced gene, and thus for symbiotic fungi colonization [58] , [59] . A RAM1/DIP1/SLR1 GRAS protein complex would then be required for the positive regulation of mycorrhizal-associated gene expression and fungi colonization. In the nodulation context, it was previously documented that NSP1 interacts with NSP2 and that this interaction is required for nodulation [16] . A NSP1/NSP2/DELLA GRAS protein complex may then positively regulate gene expression controlling rhizobial infection and nodulation. A parallel has recently been established at the molecular level between the regulation of ERN1 and RAM2 expression in response, respectively, to nodulation and mycorrhizal signals [3] , which suggests that NSP1 may be functionally equivalent to RAM1. Interestingly, DELLA proteins interact with DIP1 but not RAM1 (ref. 58 ), consistent with our results, in which we did not find interaction between DELLA proteins and NSP1, suggesting specificities in GRAS protein interactions. It remains to be tested if the DELLA/NSP2 interactions identified here are relevant for the mycorrhizal symbiosis. In this latter case, another GRAS protein different from NSP2 was identified as a DELLA interactor, suggesting that other GRAS proteins may also interact with DELLAs in the nodulation context. Our study additionally reveals that other types of NF-related transcription factors may participate in the same transcriptional complex, such as NF-YA1. Capturing the kinetics and spatial locations of these different protein interactions will be essential to determine when and where these various transcriptional complexes can be formed and on which target they act. In addition, overlaps between DELLA-transcriptional complexes recruited for rhizobial and endomyccorhizal early signalling pathways, and their relevance for the regulation of NF versus mycorrhizal signalling and the progression of symbiotic infections also remains to be determined. Materials and treatments Seeds of the M. truncatula genotypes Jemalong A17 or R108 were used in this study. The della1 (NF12399), della2 (NF4302) and della3 (NF10539) mutant lines were identified by a PCR-based reverse screening [60] of M. truncatula Tnt1 insertion population [61] , generated in the R108 genotype, at the Noble Foundation ( http://bioinfo4.noble.org/mutant/database.php ). Mutant plants were genotyped by PCR using specific primers to amplify the endogenous loci, which were also combined with the transposon-specific primer LTR4 or LTR6 ( Supplementary Table 5 for primer combinations and sequences) and backcrossed twice. The pENOD11 : GUS line was initially identified in Journet et al . [8] . Seeds were scarified and sterilized as described in Gonzalez-Rizzo et al . [18] . For in vitro nodulation experiments, germinated seeds were grown vertically on a Fahraeus medium without nitrogen [62] with 1.5% Bacto-Agar (Gibco) for 7 days in chambers at 24 °C under long-day conditions (16 h light at 150 μE light intensity/8 h dark), and then inoculated with a S. meliloti strain 1021 suspension (OD600nm=0.07) for 1 h. A derivative S . meliloti strain 2011 (ref. 63 ) carrying the pXLGD4 plasmid containing a Pro Δ ala : LACZ transcriptional fusion was additionally used for LacZ staining experiments. For in vitro pharmacological treatments, germinated seeds were grown as described above on a growth paper (Mega International, http://www.megainternational.com/index.htm ). After 2 days, the growth paper with the plants was transferred on a fresh Fahraeus medium without nitrogen, supplemented or not with increasing concentrations of GA 3 (0.001–1 μM, Sigma-Aldrich) or PAC (0.01–1 μM, Sigma-Aldrich). To generate material for real-time quantitative RT–PCR (RT–qPCR) expression analyses, twenty germinated seedlings were placed on a grid in a magenta box with a low-nitrogen liquid medium (‘i’; Blondon, 1964) and grown in a shaking incubator (125 r.p.m.) at 24 °C under long-day conditions (16 h light, 150 μE/8 h dark). After 4 days, seedlings were treated or not with 1 μM GA 3 (Sigma-Aldrich) and maintained under the same growth conditions for various incubation times (0 and 3 h). Similarly, NF purified from S. meliloti were used at 10 −9 M for 3 h, after or not, an incubation for 3 h with 1 μM GA 3 . In parallel, mock experiments were performed, by collecting untreated roots across the kinetic (0 and 3 h). Roots collected at the indicated time points were immediately frozen in liquid nitrogen. Gene expression analysis Transcriptomic data were retrieved from the M. truncatula Gene Expression Atlas (MtGEA database, http://mtgea.noble.org/v3/ ; ref. 39 ), or from the SYMBIMICS website ( https://iant.toulouse.inra.fr/symbimics/ ; ref. 41 ). For RT–qPCR experiments, total RNA was extracted from frozen roots using the RNeasy plant mini kit (Qiagen). First-strand complementary DNA (cDNA) was synthesized from 1 μg of total RNA using the Superscript II First- Strand Synthesis System (Invitrogen). Primer design was performed using Primer3 software ( http://frodo.wi.mit.edu/cgi-bin/primer3/ ). Primer combinations, showing a minimum amplification efficiency of 80%, were used in RT–qPCR experiments ( Supplementary Table 5 ). Specificity was checked both using a melting curve and by sequencing the PCR amplicons. RT–qPCR reactions were performed using the LightCycler480 SYBR Green I Master Kit on a LightCycler480 apparatus according to manufacturer's instructions (Roche). Reference genes ( RBP1 and ACTIN11 ) were selected using the geNorm software [64] . For in situ hybridizations, the protocol described in Bustos-Sanmamed et al . [65] was used on an Intavis InsituPro automat ( http://www.intavis.com/en/ ), on nodules 21 days after S . meliloti (strain 1021) inoculation. Antisense RNA probes corresponding to MtDELLA1 , MtDELLA2 and MtDELLA3 were generated. Sense and antisense RNA probes corresponding to a carbonic anhydrase (Mt CA1 ) gene were included as negative and positive controls, respectively [21] . All primers used are shown in Supplementary Table 5 . Cloning procedures For transcriptional GUS fusions, available sequences upstream of MtDELLA1 , MtDELLA2 or MtDELLA3 start codon (1,987, 1,121 or 2,431 bp, respectively) were amplified by PCR with a Pfx polymerase (Invitrogen) using primers listed in Supplementary Table 5 . PCR fragments were first cloned into the pTOPO-ENTRY/D vector (Invitrogen) and transferred using the Gateway technology (LR recombination) into the pkGWFS7 vector ( http://www.psb.ugent.be/gateway/index.php ) carrying a GUS sequence downstream of the cloning site. For della mutants complementation assays, the p MtDELLA x:DELLAx-HA constructs were obtained using the MultiSite Gateway Cloning System (Invitrogen) and the destination vector pK7m34GW [66] . For translational fusions, MtDELLA1 , MtDELLA2 or MtDELLA3 cDNAs were amplified by PCR (primer sequences shown in Supplementary Table 1 ), first cloned into the pTOPO-ENTRY/D vector (Invitrogen), and subsequently in the pK7wGF2 vector containing a p35 S-GFP cassette ( http://www.psb.ugent.be/gateway/index.php ). For 35S:HA-NF-YA1, we used the clone generated in Laloum et al . [15] , and for 35S:HA-NSP1 and 35S:HA-NSP2 in Cerri et al . [14] . For BiFC, DELLA constructs were generated using the same entry clones for LR recombination in the pGPTVII.Bar-C/NYFP vectors containing, respectively, a p35S:CYFP or a p35S:NYFP cassette ( http://www.psb.ugent.be/gateway/index.php ). For the p35S:NYFP-NF-YA1 cloning, the NF-YA1 entry clone generated in Laloum et al . [15] was recombined into the pGPTVII.Bar-NYFP vector. For p35S:NYFP-NSP1 and p35S:NYFP-NSP2, clones generated in Hirsch et al . [16] were used. For epidermal specific expression, the pFRN-RNAi vector [18] was cut with EcoRI and SmaI to remove the RNA interference (RNAi) cassette and religated with a linker containing EcoRI and KpnI sites. The p SlEXT1 promoter was excised from a pGEM-T vector [45] and cloned into these sites to generate the pFRN-p SlEXT1 vector. A della1 -Δ18 PCR fragment amplified from the pMtDELLA1 : della1 -Δ18 plasmid with Asc1- and Stu1-containing primers ( Supplementary Table 5 ) was produced and inserted into the p FRN -p SlEXT vector to generate the p SlEXT : della1 -Δ18 construct. For transactivation assay, the ARR6 promoter was removed from the pARR6-luciferase plasmid (NCBI accession number EF090414) using BamHI and NcoI restriction enzymes, and replaced by the ERN1 promoter region defined in Cerri et al . [14] , amplified from genomic DNA using BamHI- and NcoI-containing primers ( Supplementary Table 5 ). NSP1, NSP2, NF-YA1 and MtDELLA1 cDNAs were PCR-amplified and cloned in BamHI and StuI restriction sites downstream of a 35S-CaMV promoter in the pHBT plasmid (ref. 67 ; NCBI accession number EF090408). Agrobacterium rhizogenes root transformation Constructs of interest were introduced into the A. rhizogenes ARqua1 strain [68] used for M. truncatula root transformation, and transgenic roots were obtained after kanamycin (25 mg l −1 for wild-type plants, and 50 mg l −1 for the p ENOD11:GUS line) selection for 2 weeks [68] . For nodulation experiments, composite plants were transferred onto growth papers (Mega International) on a Fahraeus medium without nitrogen [62] for 1 week, and transgenic roots were inoculated as described above with a S. meliloti or a S . meliloti strain carrying a Pro Δ ala :LACZ transcriptional fusion [63] . Histochemical staining Roots from pMtDELLA:GUS composite plants or p ENOD11:GUS stable plants were collected at 0 or 1 day post inoculation (dpi) with S. meliloti or nodules 21 dpi for histochemical GUS analysis. Histochemical staining for GUS activity was performed for 3 h at 37 °C (ref. 69 ). After staining, roots or nodules were included in 3% agarose and sliced into 40 μm sections using a VT 1200S vibratome (Leica Microsystems, http://www.leica-microsystems.com/ ). When necessary, samples or sections were briefly cleared with sodium hypochlorite [69] . Roots and nodules infected by the S. meliloti strain expressing the Pro Δ ala : LACZ fusion were used for a β-galactosidase staining [62] . Stained samples were observed in bright-field light microscopy (Olympus BX53), and pictures were taken with an Olympus DP73 camera. Bimolecular fluorescence complementation For BiFC assays, the p35S:C/NYFP-MtDELLA1, p35S:C/NYFP-MtDELLA2 and p35S:C/NYFP-MtDELLA3 translational fusions were introduced into an Agrobacterium tumefaciens AGL-0 strain, and the p35S:nYFP-NSP1 (ref. 16 ), p35S:CYFP-NSP2 (ref. 16 ) and p35S:NYFP-NF-YA1 translational fusions into an A. tumefaciens GV3103 strain, and used for transient co-transformation in N. benthamiana leaves [70] . Co-IP and ChIP For Co-IP assays, the p35S: MtDELLA1 -GFP, p35S: MtDELLA2 -GFP and p35S: MtDELLA3 -GFP translational fusions were introduced into an A. tumefaciens AGL-0 strain and the p35S:HA- NSP1 (ref. 16 ), p35S:HA- NSP2 (ref. 16 ) and p35S:HA- NF-YA1 (ref. 15 ) translational fusions into an A. tumefaciens GV3103 strain. After co-transformation in N. benthamiana leaves, Co-IPs were performed using Invitrogen Protein A Dynabeads coupled with a α-GFP antibody (Roche 11814460001) [71] . Proteins were separated by SDS–polyacrylamide gel electrophoresis and detected by immunoblotting using a α-GFP antibody (AbCam Ab3277; 1/2,000) or a α-HA antibody (Sigma H6908; 1/5,000) and a α-rabbit horseradish peroxidase secondary antibody (GE Healthcare NA934; 1/10,000). Full blots are shown in Supplementary Fig. 8 . For ChIP assays, M. truncatula roots transformed with the pMtDELLA1:GFP: della1- Δ18 (ref. 32 ) construct (or GFP as a negative control) were analysed one dpi with S. meliloti . IP were performed using a α-GFP antibody (AbCam Ab6556; 1/200), and PCR with primers shown in the Supplementary Table 5 . Transient activation assays in Arabidopsis protoplasts A 3-day-old A. thaliana cell suspension was incubated in a JPL-A medium with 1% (w/v) cellulase RS (Yakult, Tokyo, Japan) and 0.2% (w/v) macerozyme R10 (Yakult) [72] . Protoplasts were collected by centrifugation and washed in the JPL medium supplemented with 0.28 M sucrose. Protoplasts (2.5 10 5 ) were transfected with 14 μg of a DNA mixture consisting of 4 μg of the pERN1:LUC construct, 9 μg of a combination of the p35S: MtDELLA1, NSP1, NSP2 and/or NF-YA1 plasmids, and 1 μg of the pUBQ10:GUS vector [67] used as an internal control to normalize the transfection efficiency. Protoplast PEG-transfections (25% (w/v) polyethylene glycol (PEG) 6,000, 450 mM mannitol, 100 mM Ca(NO 3 ) 2 were followed by two washes with a Ca(NO 3 ) 2 250 mM—JPL-A medium [72] and incubated overnight at room temperature. Protoplasts were then harvested by centrifugation (100 g , 5 min), lysed in a protoplasts lysis buffer [67] and protein extracts were clarified by centrifugation (2,000 g , 5 min). For GUS assays, protein extracts were incubated 30 min at 37 °C in a MUG substrate mix [72] and fluorescence was measured with a TECAN Infinite200 fluorimeter. For luciferase assays, protein extracts were mixed with a luciferase assay buffer (20 mM tricine pH 7.8, 5 mM MgCl 2 , 0.1 mM EDTA, 3.3 mM DTT, 270 μM CoA, 500 μM luciferin and 500 μM ATP) and luminescence was immediately measured using a TECAN Infinite200 luminometer. Statistical analyses Statistical analyses were performed with non-parametric tests, Mann–Whitney when n =2 independent samples, and Kruskal and Wallis when n >2 independent samples. Data availability The authors declare that all data supporting the findings of this study are available within the article and its Supplementary Information Files or are available from the corresponding author upon request. How to cite this article: Fonouni-Farde, C. et al . DELLA-mediated gibberellin signalling regulates Nod factor signalling and rhizobial infection. Nat. Commun. 7:12636 doi: 10.1038/ncomms12636 (2016).